Synthesis of acetic acid via methanol hydrocarboxylation with CO2and H2 Acetic acid is an important bulk chemical that is currently produced via methanol carbonylation using fossil based CO. Synthesis of acetic acid from the renewable and cheap CO 2 is of great importance, but state of the art routes encounter difficulties, especially in reaction selectivity and activity. Here we report a route to produce acetic acid from CO 2 , methanol and H 2 . The reaction can be efficiently catalysed by Ru–Rh bimetallic catalyst using imidazole as the ligand and LiI as the promoter in 1,3-dimethyl-2-imidazolidinone (DMI) solvent. It is confirmed that methanol is hydrocarboxylated into acetic acid by CO 2 and H 2 , which accounts for the outstanding reaction results. The reaction mechanism is proposed based on the control experiments. The strategy opens a new way for acetic acid production and CO 2 transformation, and represents a significant progress in synthetic chemistry. Acetic acid is an important bulk chemical [1] , [2] that is currently produced via methanol carbonylation (CH 3 OH+CO→CH 3 COOH), such as Monsanto process [3] . CO 2 is a greenhouse gas [4] and its fixation into value-added chemicals is highly desirable for a sustainable society [5] . So far, CO 2 has been utilized to synthesize various chemicals [6] , [7] , [8] , [9] , [10] , [11] , such as alcohols, urea, carbonates, polymers and carboxylic acids. In the field of carboxylic acids syntheses using CO 2 , major advance has been focused on hydrogenating CO 2 into formic acid or its derivatives [12] , [13] , [14] , [15] , [16] , [17] , [18] , [19] and hydrocarboxylating unsaturated hydrocarbons or nucleophiles into fine chemicals [20] , [21] , [22] , [23] , [24] . Synthesis of acetic acid utilizing CO 2 is of great importance, but is challenging. The reported routes suffer from obvious disadvantages, such as low selectivity, low activity, higher reaction temperature and use of expensive and/or toxic reactants [25] , [26] , [27] , [28] , [29] . For example, acetic acid could form slowly with low selectivity when CO 2 was reduced by iron nanoparticles [25] . Synthesis of acetic acid from CO 2 and CH 4 is thermodynamically unfavourable, thus high temperature is required and the acetic acid yield is very low [26] , [27] . Trace acetic acid in CO 2 hydrogenation was detected where CO accounted for 96% of the total product [28] . When methyl iodide (CH 3 I), CO 2 and H 2 were used as reactants acetic acid was formed at low rate and selectivity (acetic acid 10.7%, CO 58.4%, and CH 4 30.9%) [29] . In addition, the reactant CH 3 I is toxic and expensive. Here we show a protocol to produce acetic acid from CO 2 , methanol and H 2 ( Fig. 1 ). The reaction could proceed very efficiently by homogeneous catalysis under mild condition. Interestingly, the CO 2 (not via CO) participates in acetic acid formation with H 2 , accounting for the outstanding reaction results. The strategy represents a significant progress in synthetic chemistry. Because the reported routes of hydrocarboxylation use other substrates, such as alkenes, alkynes, arenes and/or organic halides, and the metallic reducing agents are generally utilized [20] , [21] , [22] , [23] , [24] . This work opens a practical way to fix CO 2 into bulk chemicals using easily available and cheap feedstocks, which is a promising countermeasure for mankind to solve the ever-increasing crisis in environment and resources. 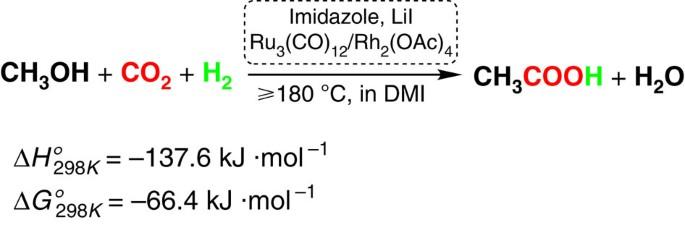Figure 1: Synthesis of acetic acid by reaction of methanol with CO2and H2. In the reaction CO2participates in acetic acid formation with H2, and does not via CO. Figure 1: Synthesis of acetic acid by reaction of methanol with CO 2 and H 2 . In the reaction CO 2 participates in acetic acid formation with H 2 , and does not via CO. Full size image Catalytic system for acetic acid synthesis The target reaction was catalysed effectively by Ru–Rh bimetallic catalyst using imidazole as the ligand and LiI as the promoter in 1,3-dimethyl-2-imidazolidinone (DMI) at milder conditions ( Table 1 ). Acetic acid was the predominant product and other products being negligible in the reaction solution ( Supplementary Fig. 1a ). The turnover frequency (TOF) of acetic acid reached 30.8 h −1 and the yield of acetic acid based on methanol was 70.3% (Entry 1). The rest of the methanol was converted into CH 4 . Very interestingly, the CO was hardly detectable in the gaseous sample ( Supplementary Fig. 1b ). Table 1 Methanol hydrocarboxylation using different catalytic systems. Full size table The ligand was crucial to the catalytic performance. Without ligand, the catalyst was unstable with much lower activity and selectivity (Entry 2). We also tried other ligands, but the results were not satisfactory (Entries 3–6). So imidazole was the suitable ligand for the reaction. The high efficiency of imidazole in this reaction should be due to its good coordination capability with the active center, which will be discussed in detail in the following paragraph. The promoter was also indispensable in this reaction. Without promoter, no acetic acid was formed and the catalyst was unstable (Entry 7). When the promoters with other cations (Na + , K + and Sn 4+ ) or anions (Cl − and Br − ) were utilized, the results were poor (Entries 8–13). Therefore, LiI was the best promoter in catalysing the target reaction. The better performance of lithium cation may be due to its stronger Lewis acidity and proper ion size, which could render appropriate coordination sites during the reaction. The superiority of the iodide anion could be attributed to its stronger nucleophilicity, which would facilitate the C–C bond formation in the generation of acetic acid. We tested Ru 3 (CO) 12 as single catalyst but no acetic acid formed (Entry 14). When we tried Rh 2 (OAc) 4 separately, acetic acid formed at a lower rate (Entry 15). Thus, Rh complex was the major catalyst and Ru complex was the co-catalyst. We have combined Rh 2 (OAc) 4 with other Ru compounds, such as RuO 2 or Ru(PPh 3 ) 3 Cl 2 , but the reaction results were poor (Entries 16, 17). We also combined Ru 3 (CO) 12 with other Rh compounds, such as RhCl 3 ·3H 2 O or Rh(CO)H 2 (PPh 3 ) 3 , but the efficiencies were also not satisfactory (Entries 18, 19). Obviously, synergistic effect existed between the Ru–Rh catalysts in accelerating the reaction (Entry 1). The superiority of the Ru 3 (CO) 12 /Rh 2 (OAc) 4 in producing acetic acid could be ascribed to their fitness in triggering the synergistic effect. The solvent effect is also important for the reaction. On the basis of Ru 3 (CO) 12 /Rh 2 (OAc) 4 , imidazole and LiI, other solvents were tested, but the catalytic performances were poor (Entries 20–24). When other solvents, such as DMF, tetrahydrofuran, cyclohexane and water, were used, the metal complex decomposed during the reaction and evident black precipitates were observed. The results indicate that DMI could stabilize the catalyst. As a weak Lewis base, DMI may also help to absorb and activate acidic CO 2 . Moreover, the DMI is stable under H 2 atmosphere and the generation of acetic acid from acetate in Rh 2 (OAc) 4 was excluded because the reaction did not occur when only H 2 was used as the reactant (Entry 25). Hence, the catalytic system consisting of Ru 3 (CO) 12 , Rh 2 (OAc) 4 , imidazole, LiI, and DMI was the best for the target reaction. Effect of reaction parameters On the basis of the optimized catalytic system, we studied the effects of reaction temperature, pressure and dosage of each catalyst component on the reaction. 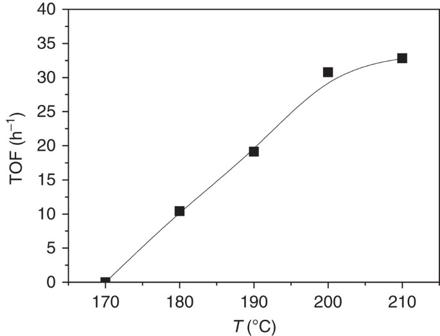Figure 2: The TOF of acetic acid at different temperatures. Condition: 40 μmol Ru3(CO)12and 40 μmol Rh2(OAc)4(based on metals), 0.75 mmol imidazole, 3 mmol LiI, 2 ml DMI, 12 mmol MeOH, 4 MPa CO2and 4 MPa H2(at room temperature), and 12 h. TOF denotes moles of acetic acid produced per mole of Rh catalyst per hour in the steady state. Figure 2 shows the TOF of acetic acid at different temperatures. The acetic acid was not detectable when the reaction was carried out at 170 °C, and it emerged with remarkable amount when the temperature was elevated to 180 °C. The activity grew steadily with the increase of temperature until 200 °C. The TOF of acetic acid at 200 °C reached 30.8 h −1 and increased slowly when the temperature was further increased. Figure 2: The TOF of acetic acid at different temperatures. Condition: 40 μmol Ru 3 (CO) 12 and 40 μmol Rh 2 (OAc) 4 (based on metals), 0.75 mmol imidazole, 3 mmol LiI, 2 ml DMI, 12 mmol MeOH, 4 MPa CO 2 and 4 MPa H 2 (at room temperature), and 12 h. TOF denotes moles of acetic acid produced per mole of Rh catalyst per hour in the steady state. Full size image The results in Fig. 2 suggest that 200 °C is a suitable temperature. We further studied the effects of other parameters on the reaction at this temperature, and the results are given in Table 2 . The pressure of the reaction gases (CO 2 and H 2 ) evidently affected the reaction. At fixed ratio of CO 2 and H 2 (1:1), the yield of acetic acid increased markedly as the total pressure was raised from 2 to 10 MPa (Entries 1–5). At a fixed total pressure of 8 MPa, the ratio of CO 2 and H 2 also influenced the reaction and highest yield of acetic acid was obtained at the ratio of 1:1 (Entries 4, 6, 7). In the absence of CO 2 or H 2 , the reaction did not occur (Entries 8, 9). Hence both CO 2 and H 2 are necessary for the formation of acetic acid. These results demonstrated that acetic acid was not generated from the CO in Ru 3 (CO) 12 via methanol carbonylation, and DMI was stable at the reaction condition. Table 2 Effect of reaction parameters on methanol hydrocarboxylation. Full size table The dosages of imidazole and LiI also influenced the reaction significantly. The yield of acetic acid was the highest when 750 μmol of imidazole was used (Entries 4, 10, 11), and the highest yield occurred at LiI dosage of 3 mmol (Entries 4, 12, 13). The results indicate that excess amount of imidazole or LiI was not favourable to the reaction. The main reason may be that the active sites were occupied by the excess imidazole or iodide anions due to their good coordination capability, and the reaction was inhibited accordingly. The atom ratio of the Ru and Rh also affected the yield of the reaction. At the same total amount of Ru and Rh (80 μmol), 40 μmol Ru+40 μmol Rh gave the highest yield of acetic acid (Entries 4, 14, 15). As expected, the total yield of acetic acid increased with increasing catalyst dosage (Entries 4, 16, 17), but it was less sensitive when the amount of catalyst was large enough. The above results reveal that the reaction condition in Entry 1 of Table 1 was the optimal. Recyclability To study the reusability of the catalytic system, the acetic acid generated in the reaction system was removed in a vacuum oven at 85 °C for 5 h, and GC analysis showed that the acetic acid remained in the reactor was negligible after the evacuation process, then the catalytic system was used directly for the next run. The results indicated that the catalytic activity did not change considerably after five cycles and the TON of acetic acid reached 1,022 in the five cycles. ( Fig. 3 ). 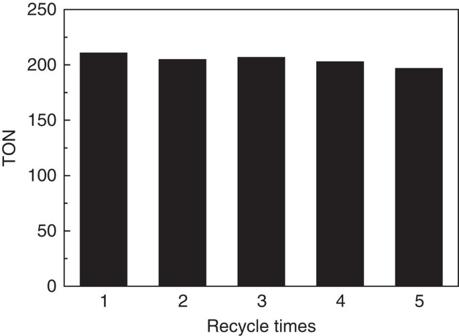Figure 3: The results of the recycling test. Condition: 40 μmol Ru3(CO)12and 40 μmol Rh2(OAc)4(based on metals), 0.75 mmol imidazole, 3 mmol LiI, 2 ml DMI, 12 mmol MeOH, 4 MPa CO2and 4 MPa H2(at room temperature), 200 °C, and 12 h. TON denotes moles of acetic acid produced per mole of Rh catalyst. Figure 3: The results of the recycling test. Condition: 40 μmol Ru 3 (CO) 12 and 40 μmol Rh 2 (OAc) 4 (based on metals), 0.75 mmol imidazole, 3 mmol LiI, 2 ml DMI, 12 mmol MeOH, 4 MPa CO 2 and 4 MPa H 2 (at room temperature), 200 °C, and 12 h. TON denotes moles of acetic acid produced per mole of Rh catalyst. 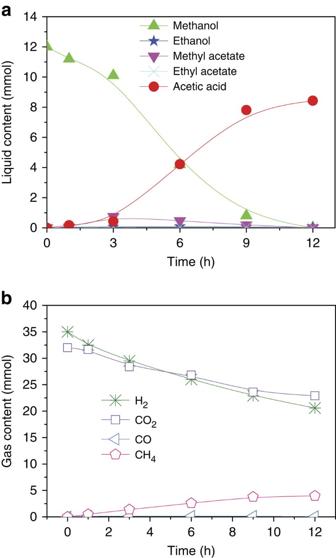Figure 4: Time course of the methanol hydrocarboxylation. (a) Liquid content, (b) gas content. Condition: 40 μmol Ru3(CO)12and 40 μmol Rh2(OAc)4(based on metals), 0.75 mmol imidazole, 3 mmol LiI, 2 ml DMI, 12 mmol MeOH, 4 MPa CO2and 4 MPa H2(at room temperature), 200 °C. Full size image Time course of the reaction Figure 4 presents the time course of the reaction. The amount of acetic acid increased slowly at the beginning (0–3 h) mainly because the acetic acid reacted with methanol to form methyl acetate. After that time the amount of acetic acid increased steadily (3–9 h). The reaction slowed down when methanol feedstock was gradually used up (9–12 h). As expected, with consumption of methanol, the methyl acetate formed initially was converted into acetic acid because of reverse esterification. The CO 2 consumption directly correlated with the production of acetic acid. The amount of CH 4 generated in the reaction was minor. Surprisingly, in the whole process, CO was nearly undetectable and alcohols formation was negligible. Figure 4: Time course of the methanol hydrocarboxylation. ( a ) Liquid content, ( b ) gas content. Condition: 40 μmol Ru 3 (CO) 12 and 40 μmol Rh 2 (OAc) 4 (based on metals), 0.75 mmol imidazole, 3 mmol LiI, 2 ml DMI, 12 mmol MeOH, 4 MPa CO 2 and 4 MPa H 2 (at room temperature), 200 °C. Full size image Role of the imidazole To understand the above results, we studied the hydrogenation of CO using the catalytic system. The results showed that plenty of alcohols and CH 4 were generated, and imidazole had no obvious impact on the reaction ( Supplementary Figs 2 and 3 ). When we tried CO 2 hydrogenation without imidazole, considerable amounts of CO, alcohols and CH 4 were formed in the reaction ( Supplementary Fig. 4 ). Because CO is a well-known intermediate in CO 2 hydrogenation to generate alcohols and alkanes [30] , we could deduce that in the absence of imidazole the CO 2 was firstly transformed into CO, then alcohols and CH 4 were produced via CO hydrogenation. However, CO and liquid product formed were negligible when the imidazole was used in the CO 2 hydrogenation reaction ( Supplementary Fig. 5 ). Hence, we conclude that the imidazole inhibited hydrogenation of CO 2 into CO, which is the origin for the excellent selectivity of acetic acid in this work. As we have mentioned in the former paragraph, the imidazole also played a key role in catalytic activity and stability. The X-ray photoelectron spectroscopy study revealed the facile coordination of imidazole with the Ru and Rh catalysts, which accounted for the role of imidazole in the reaction ( Supplementary Fig. 6 ). Reaction pathway Production of acetic acid from CO and methanol, that is, methanol carbonylation, is a well-known reaction [3] . So there are two possible pathways of acetic acid synthesis from CO 2 , methanol and H 2 . The first is the CO pathway, that is, the CO 2 was hydrogenated to CO, then acetic acid was formed by methanol carbonylation. The second is the CO 2 pathway, namely, the methanol was hydrocarboxylated into acetic acid by CO 2 and H 2 . All the above experimental results support the second pathway. To get further evidence to support the above argument, we studied the time course of the reaction of CO, methanol and H 2 ( Fig. 5 ). At the beginning, methanol was mostly homologated into ethanol by CO and H 2 , accompanying with gradual accumulation of CO 2 because CO 2 is a common byproduct in the methanol homologation, especially in the presence of amines [31] . At 6 h, CO in the reactor decreased to 3.5 mmol and CO 2 increased to 12.5 mmol accordingly. At this point, the ethanol generation ceased and minor acetates formed. With time going on, the CO 2 played a key role in the reaction. After 9 h, the CO 2 content dropped obviously and considerable acetic acid and acetates emerged accordingly. These results rule out the possibility of first pathway (via CO). The CO 2 pathway was further confirmed by tracer experiments using CH 3 OD, CH 3 18 OH and 13 CH 3 OH, respectively ( Supplementary Figs 7, 8 and 9 ). To our knowledge, this is the first work on methanol hydrocarboxylation with CO 2 and H 2 . It is an important contribution to synthetic chemistry. 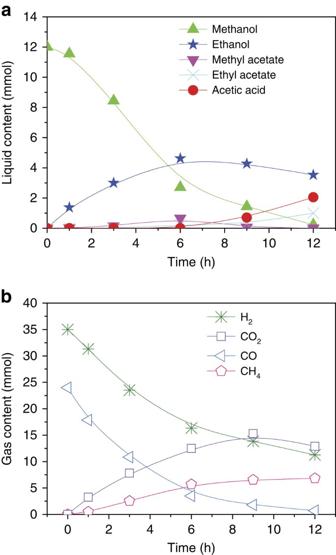Figure 5: Time course of the reaction of methanol with CO and H2. (a) Liquid content, (b) gas content. Condition: 40 μmol Ru3(CO)12and 40 μmol Rh2(OAc)4(based on metals), 0.75 mmol imidazole, 3 mmol LiI, 2 ml DMI, 12 mmol MeOH, 4 MPa CO and 4 MPa H2(at room temperature), 200 °C. Figure 5: Time course of the reaction of methanol with CO and H 2 . ( a ) Liquid content, ( b ) gas content. Condition: 40 μmol Ru 3 (CO) 12 and 40 μmol Rh 2 (OAc) 4 (based on metals), 0.75 mmol imidazole, 3 mmol LiI, 2 ml DMI, 12 mmol MeOH, 4 MPa CO and 4 MPa H 2 (at room temperature), 200 °C. Full size image On the basis of all the results above, we proposed the possible mechanism of the reaction ( Fig. 6 ). There are five major steps in the reaction cycle. First, methanol is in situ converted into methyl iodide, which is similar to the Monsanto process. (Step 1). It is known that CH 3 I could form spontaneously from methanol and iodine compounds at elevated temperature [32] , which would be promoted by the Lewis acidic cation (Li + ) [33] . The CH 3 I is a commonly used promoter or intermediate in organic reactions [3] , [8] , [32] , [33] . The tracer experiments using CH 3 OD and CH 3 18 OH affirmed that the OH broke away from CH 3 OH during the reaction, supporting the formation of CH 3 I ( Supplementary Figs 7 and 8 ). The NMR spectra of the reaction solution using 13 CH 3 OH as reactant ( Supplementary Fig. 10 ) also verified that the CH 3 group of methanol is transferred into the acetic acid molecule, which is consistent with the proposed mechanism. Secondly, CH 3 Rh*I was formed via oxidative addition of CH 3 I to the active Rh species (Rh*) (Step 2). The oxidative addition is a basic step in organic synthesis and has been well studied [3] , [32] , [33] . In addition, the tracer experiment and NMR spectra using 13 CH 3 OH supported the transfer of CH 3 group during the reaction ( Supplementary Figs 9 and 10 ). The third step was the insertion of CO 2 into CH 3 Rh*I to form CH 3 COORh*I (Step 3). Rh catalyst was responsible for generating acetic acid (Entry 15 of Table 1 ). The insertion of CO 2 into Rh-alkyl bond (including CH 3 –Rh bond) has been well studied [34] , which could be accelerated by enhancing the electron density of the Rh atom. The coordination with imidazole may increase the electron density of the Rh*, which explains the role of imidazole in facilitating the catalytic activity. During the insertion of CO 2 into the CH 3 –Rh bond, the CH 3 COORh*I formed and the O atom of the C-O adsorbed on the catalyst before further reaction [34] . Next step was reductive elimination of acetic acid from the CH 3 COORh*I in the presence of H 2 , which was promoted by the active Ru species (Ru*) (Step 4). The tracer experiment and NMR spectra using 13 CH 3 OH indicated that the CH 3 group of methanol finally entered into the acetic acid molecule ( Supplementary Figs 9 and 10 ). The tracer experiments using CH 3 OD affirmed that the H in the COOH group of acetic acid was from the reactant H 2 ( Supplementary Fig. 7 ). The catalytic data showed that acetic acid generation was remarkably promoted by the Ru catalyst (Entries 1, 15 of Table 1 ). The promoting effect of Ru complex on hydrogenating intermediate into product has been reported in other Rh catalysed reactions [35] . Finally, the LiOH and HI generated in situ neutralized spontaneously to form LiI and H 2 O (Step 5). At this time, all the catalytic species were regenerated for the next cycle. 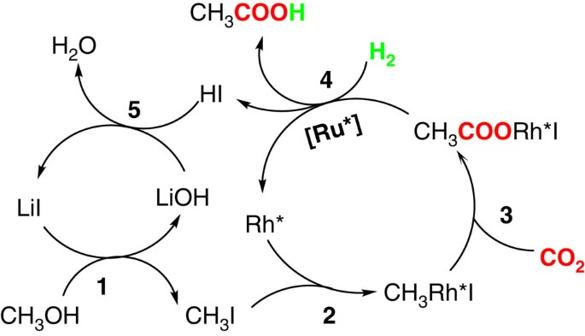Figure 6: Proposed mechanism. The Ru* and Rh* represent the active Ru and Rh species in the reaction, respectively. Figure 6: Proposed mechanism. The Ru* and Rh* represent the active Ru and Rh species in the reaction, respectively. Full size image In summary, we have developed a route of acetic acid synthesis from methanol, CO 2 and H 2 . The reaction is efficiently promoted by Ru–Rh bimetallic catalyst. The acetic acid can be generated in large amount at above 180 °C, and the TON of acetic acid exceeds 1,000 after five cycles. The ligand imidazole plays a key role for the high catalytic stability, activity and selectivity of the catalyst. The reaction does not proceed via CO pathway. This route has great potential of application because cheap, easily available starting materials are used and the efficiency is high. Future work is to study the detailed reaction mechanism and design catalytic systems of better performance for industrial application. Chemicals Ruthenium carbonyl (Ru 3 (CO) 12 , 98%) and potassium bromide (KBr, 99.9%) were purchased from Adamas Reagent, Ltd. Ruthenium(IV) oxide (RuO 2 , 99.9%, metal basis), Dichlorotris (triphenylphosphine) ruthenium(II) (Ru(PPh 3 ) 3 Cl 2 , 97%), Carbonylhydridotris (triphenylphosphine)rhodium(I) (Rh(CO)H 2 (PPh 3 ) 3 , Rh>10%), Rhodium(III) chloride hydrate (RhCl 3 ·3H 2 O, Rh>38.5%), imidazole (99%), lithium bromide (LiBr, 99%), lithium iodide (LiI, 99.95%), sodium iodide (NaI, 99.5%), potassium iodide, (KI, 99.9%), Tin(IV) iodide (SnI 4 , 99.998%), Triphenylphosphine (PPh 3 , 99%), 2,2′-Bipyridine (99%) and Bis(triphenylphosphoranylidene) ammonium chloride (PPN–Cl, 97%) were obtained from Alfa Aesar China Co., Ltd. Rhodium acetate dimer (Rh 2 (OAc) 4 ), lithium chloride (LiCl, 98%) and 1,3-Dimethyl-2-imidazolidinone (DMI, 99%) were purchased from TCI Shanghai Co., Ltd. N -Methyl-2-pyrrolidone (NMP, 99.5%), N , N -dimethylformamide (DMF, 99.5%), cyclohexane (99.5%) and pyridine (99%) were provided by Sinopharm Chemical Reagent Co., Ltd. Methanol (99.5%), tetrahydrofuran (A.R. grade) was obtained from Beijing Chemical Company. Toluene (99.8%, HPLC) was obtained from Xilong Chemical Co., Ltd. Methanol– 13 C ( 13 CH 3 OH, 99 atom% 13 C) and Methanol– 18 O (CH 3 18 OH, 95 atom% 18 O) were purchased from Sigma-Aldrich Co. LLC. Methanol–D 1 (CH 3 OD, 99.5 atom% D) was provided by Beijing InnoChem Science & Technology Co., Ltd. The CO 2 (99.99%) and H 2 (99.99%) were purchased Beijing Analytical Instrument Company. Catalytic reaction All the reactions were conducted in a 16 ml Teflon-lined stainless steel batch reactor equipped with a magnetic stirrer. The inner diameter of the reactor was 18 mm. In a typical experiment, known amounts of Ru and/or Rh catalysts, imidazole or another ligand, LiI or another promoter, methanol or ( 13 CH 3 OH, CH 3 18 OH or CH 3 OD if used), and 2 ml DMI or another solvent were loaded sequentially into the reactor. The reactor was purged two times with CO 2 of 1 MPa in ice-water. At room temperature, CO 2 in the cylinder was charged into the reactor to desired pressure, and the inlet valve of CO 2 was closed. Then H 2 was charged into the reactor until suitable total pressure was reached. The reactor was placed in an air bath of constant temperature, and the magnetic stirrer was started at 800 r.p.m. After reaction, the reactor was cooled in an ice-water bath for 1 h, the residual gas was released slowly and collected in a gasbag. The liquid mixture was analysed by GC (Agilent 7890B) equipped with a flame ionization detector and an HP-5 capillary column (0.32 mm in diameter, 30 m in length) using toluene as the internal standard. Identification of the liquid products was done using a GC–MS (SHIMADZU-QP2010) as well as by comparing the retention times of the standards in the GC traces. The yields of the products were calculated from the GC data. The gaseous samples were analysed using a GC (Agilent 4890D) equipped with a TCD detector and a packed column (Carbon molecular sieve TDX-01, 3 mm in diameter and 1 m in length) using Argon as the carry gas. Recycling test After reaction, the reactor was cooled down using an ice bath and the residual gas was released. The amount of product was determined as discussed above. Then the acetic acid formed and the unreacted methanol in the reactor were removed in a vacuum oven at 85 °C for 5 h. GC analysis confirmed the complete removal of the acetic acid at this condition. The catalytic system (catalyst+promoter+DMI) was used directly for the next run. How to cite this article: Qian, Q. et al . Synthesis of acetic acid via methanol hydrocarboxylation with CO 2 and H 2 . Nat. Commun. 7:11481 doi: 10.1038/ncomms11481 (2016).